Enantioselective synthesis of [4]helicenes by organocatalyzed intermolecular C-H amination Catalytic asymmetric synthesis of helically chiral molecules has remained an outstanding challenge and witnessed fairly limited progress in the past decades. Current methods to construct such compounds almost entirely rely on catalytic enantiocontrolled fused-ring system extension. Herein, we report a direct terminal peri -functionalization strategy, which allows for efficient assembling of 1,12-disubstituted [4]carbohelicenes via an organocatalyzed enantioselective amination reaction of 2-hydroxybenzo[ c ]phenanthrene derivates with diazodicarboxamides. The key feature of this approach is that the stereochemical information of the catalyst could be transferred into not only the helix sense but also the remote C-N axial chirality of the products, thus enabling the synthesis of [4]- and [5]helicenes with both structural diversity and stereochemical complexity in good efficiency and excellent enantiocontrol. Besides, the large-scale preparations and representative transformations of the helical products further demonstrate the practicality of this protocol. Moreover, DFT calculations reveal that both the hydrogen bonds and the C-H---π interactions between the substrates and catalyst contribute to the ideal stereochemical control. As screw-shaped compounds formally derived from ortho -annulated aromatic and/or hetero-aromatic rings, helically chiral molecules have fascinated synthetic chemists for more than 100 years owing to their esthetic architectures and unique chiroptical properties [1] , [2] , [3] , [4] , [5] , [6] . Tremendous efforts have been devoted to developing the methodologies for the synthesis of enantiomerically pure helicenes, which have been demonstrated in the past decades to be highly promising for application in diverse fields, such as asymmetric catalysis [7] , [8] , [9] , molecular recognition [10] , [11] , [12] , molecular machines [13] , [14] , material sciences [15] , [16] , [17] , and some biologically active agents [18] , [19] . Incipiently, substrate-controlled diastereoselective cyclisation reactions were employed to induce the screw sense of the helicenes [20] , [21] , [22] , [23] , [24] , [25] , [26] , [27] . However, the utilizing of chiral auxiliaries or tethers inevitably led to tedious and complicated preparation of enantiomerically enriched starting materials and high economic cost. In this regard, catalytic asymmetric protocols with high levels of stereocontrol are particularly alluring, but have proven to be extremely challenging. While approaches to optically pure point-chiral [28] and axially chiral compounds [29] , [30] have mushroomed enormously in the past decades, catalytic enantioselective synthesis of helicenes [31] , [32] is still in its infancy, and corresponding literatures reported to date have been fairly limited (Fig. 1a ). Progress in this field mainly comes from transition-metal-catalyzed [2 + 2 + 2] cycloadditions [33] , [34] , [35] , [36] , [37] , [38] , [39] , [40] , [41] , [42] and intramolecular hydroarylation of alkynes [43] , [44] , [45] , [46] , [47] , [48] , [49] , [50] , [51] . Complementally, sporadic transition-metal-catalyzed other approaches [52] , [53] , [54] , such as V-catalyzed oxidative coupling of polycyclic phenols and Rh-catalyzed enantioselective C-H activation/annulation process of 1-aryl isoquinoline derivatives and alkynes were reported by Sasai and You, respectively. Besides, the rare examples of organocatalyst-mediated cycloadditions were also documented to be efficient to access enantiomerically enriched helicenes [55] , [56] , [57] , [58] . Especially, it is noteworthy that during the preparation of this manuscript, Baudoin and co-workers reported a Pd-catalyzed enantioselective intramolecular C-H arylation for access to lower carbo[ n ]helicenes [59] , groups of Yang and Li independently published the chiral phosphoric acid catalyzed enantioselective Povarov reaction/oxidative aromatization process to allow for the synthesis of azahelicenes [60] , [61] . However, despite these pioneering and elegant works, nearly all the approaches mentioned above utilized a strategy of extending fused-ring systems through stereoselective cyclizations to construct configurationally stable helicenes (Fig. 1b–I ) [33] , [34] , [35] , [36] , [37] , [38] , [39] , [40] , [41] , [42] , [43] , [44] , [45] , [46] , [47] , [48] , [49] , [50] , [51] , [52] , [53] , [54] , [55] , [56] , [57] , [58] , [59] , [60] , [61] . The scarcity of complementary assembly strategies has significantly hindered the on-demand synthesis of helicenes or helicene-like molecules through catalytic enantioselective methods. Therefore, the exploration of more innovative and practical concepts for obtaining optically pure helicenes with a wide structural diversity is highly desired. Fig. 1: Background introduction and our strategy for synthesizing optically pure helicenes. a The research status of catalytic enantioselective synthesis of chemicals with different types of chiralities. b Strategies for the enantioselective synthesis of hetero- and carbohelicenes. TM transition metal. Full size image It should be noted that besides π-conjugated scaffold extension through arene formation, terminal peri -functionalization of the choreographed substrates could also generate configurationally stable [4]- and [5]helicenes. However, such a tactic has hitherto not been applied in the catalytic enantioselective synthesis of functionalized helicenes and their heteroanalogues (Fig. 1b-II ), which might arise from three reasons: (1) there is few or no appropriate and available substrate; (2) the large steric hindrance caused by terminal ring makes it difficult to install a substituent group at the fjord region of the helical precursors; (3) unlike building stereogenic centers, the control of helical chirality is more challenging because it is a phenomenon of nanoscale, which calls for the pursuit or design of rational catalyst to obtain satisfactory enantioselectivity. To realize this vision, benzo[ c ]phenanthren-2-ol 1 with a substituent at its 12-position, in which the hydroxyl group could function as both a directing group and a binding site, was designed and synthesized (Fig. 2 ). We speculated that diverse functional groups could be incorporated at the 1-position in a catalytic helicoselective fashion by utilizing the nucleophilicity of the enol tautomer of substrate 1 , thereby increasing the barrier to enantiomerization and giving access to enantioenriched 1,12-disubstituted [4]helicenes. If such an endeavor meets with success, a series of highly functionalized helicene molecules that had previously been unexploited or inaccessible would be easily assembled via an intermolecular electrophilic aromatic substitution reaction. Fig. 2: Diverse synthesis of compounds with different chiralities via catalytic enantioselective amination reactions of polycyclic phenols. a Previous works: construction of axially and centrally chiral compounds by Friedel-Crafts and dearomative aminations. b This work: construction of helically chiral molecules by developing a terminal peri -amination strategy. CPA chiral phosphoric acid. Full size image For this purpose, we speculated that highly reactive azo-compound [62] might be a suitable electrophile to realize the functionalization of highly steric-hindered fjord-type area of polycyclic phenol 1 . To the best of our knowledge, catalytic asymmetric amination reaction of phenols with azo-compounds represents one of flexible and versatile protocols for preparing functionalized molecules with different stereogenic elements. For example, groups of Jørgensen and Tan independently realized the catalytic asymmetric synthesis of C-N axially chiral compounds by employing a direct C-N axis construction strategy and a desymmetrisation strategy, respectively (Fig. 2a-I ) [63] , [64] , [65] , [66] . Besides, You group, Luan group, and Pan group successively reported the catalytic asymmetric assembling of aza-quaternary carbon centers by utlizing dearomative amination reactions of α-substituted β - naphthols with either azodicarboxylates or diazodicarboxamides (Fig. 2a-II ) [67] , [68] , [69] . However, despite these conspicuous progresses, the applications of similar chemical processes in helicenes synthesis have not yet been reported, even in a non-helicoselective version. To further extend the potential of Friedel-Crafts amination reactions in asymmetric synthesis and enrich the synthetic strategies of enantioenriched helicenes, we reported herein an enantioselective terminal peri -amination strategy for the efficient synthesis of configurationally stable [4]- and [5]helicenes (Fig. 2b ). Optimization of reaction conditions Initially, the amination reaction of 12-methylbenzo[ c ]phenanthren-2-ol 1a and diazodicarboxamide 2a was selected as model reaction to examine the feasibility of our concept. Considering the extraordinary performance of bifunctional organocatalysts in asymmetric catalysis [70] , [71] , we envisage that a double-activation mode via H-bonding interactions could be applied to promote the depicted pathway and control the stereochemistry. 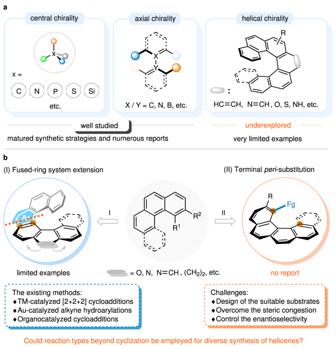Fig. 1: Background introduction and our strategy for synthesizing optically pure helicenes. aThe research status of catalytic enantioselective synthesis of chemicals with different types of chiralities.bStrategies for the enantioselective synthesis of hetero- and carbohelicenes. TM transition metal. Accordingly, typical Takemoto thiourea catalyst C1 was first employed to drive the current reaction, and pleasingly, furnished the desired [4]helicene 3a in 41% yield with 67.5:32.5 er at −50 °C (Table 1 , entry 1). As expected, the C-H amination of 1a indeed brought a sufficient increase in the energy barrier of racemization, leading to the formation of a pair of enantiomers that were configurationally stable enough and not interconvertible at room temperature. Motivated by this result, commercially available cinchona alkaloid-derived thiourea C2 and squaramide C3 , as well as ( S , S )−1,2-cyclohexanediamine-derived thioureas C4 and C5 were evaluated to further improve the enantioselectivity (entries 2-5). However, only C4 delivered a slightly increased er value. In the light of relatively larger size of helical topology, it was conjectured that extending the steric hindrance group of the catalyst might avail to the long-range control of enantioselectivity. With this in mind, catalyst C6 bearing a 1-pyrenyl substituent was synthesized and provided a significantly improved enantioselectivity (entry 6, 86:14 er). The subsequent solvent screening revealed a preference for THF (entries 7–9). When the concentration and scale of the reaction mixtures were increased, the same excellent outcome was obtained (entry 11, 45% yield, 96.5:3.5 er). Table 1 Optimization of the reaction conditions a Full size table Substrate scope Having established the optimal reaction conditions, we sought to investigate the substrate scope and limitations of this intermolecular amination reaction. A variety of diazodicarboxamides 2 were examined in combination with 12-methylbenzo[ c ]phenanthren-2-ol 1a (Fig. 3 ). Either electron-donating or electron-withdrawing groups at the para -position of the phenyl ring were all compatible with this protocol, affording the corresponding 1,12-disubstituted [4]helicenes in high yields and enantioselectivities ( 3b - 3j , 37-46% yield, 95.5:4.5-98:2 er). Changing the position of methyl substituent on the phenyl ring had no apparent effect on the reaction results ( 3k - 3l ). Pleasingly, the reactions of diazodicarboxamides with a disubstituted phenyl ring occurred in satisfactory yields and enantioselectivities ( 3m - 3p ). Only in the case of 3n was a relatively diminished yield (28%) observed, probably resulting from rapid decomposition of substrate 2n . Moreover, diazodicarboxamide bearing a bulkier naphthalene group also worked well ( 3q ). Importantly, the substituent of substrate 2 has not to be aromatic in nature; alkyl-substituted substrates, such as those with benzyl, n -hexyl and cyclohexyl, were all smoothly converted to the desired enantioenriched [4]helicenes with excellent outcomes ( 3r - 3t , 38–44% yield, 96:4-98:2 er), which further highlighted the compatibility of this transformation. Fig. 3: Substrate scope with respect to diazodicarboxamides. Reaction conditions: 0.2 mmol 1a (1.0 equiv), 0.1 mmol 2 (0.5 equiv), and 5 mol% C6 in THF (1.0 mL) at −50 °C. Isolated yields based on 1a are shown. The er values were determined by HPLC analysis using a chiral stationary phase. Full size image Next, we targeted the exploration of substrate scope with respect to 2-hydroxybenzo[ c ]phenanthrenes 1 (Fig. 4 ). The effect of substituents at position 12 was first examined. Besides methyl, ethyl and relatively bulky isopropyl groups were all well tolerated, and the corresponding amination products were obtained in excellent yields and enantioselectivities ( 3u, 3v ). Substitutions at the 10 and 11 positions of the terminal aromatic ring with a fluorine atom or a methyl group saw a slight decrement in enantioselectivities ( 3w - 3y , 85:15-92.5:7.5 er) with increased steric hindrance effect, but led to consistently excellent chemical yields (45-49% yield). Such a decline in enantioselectivity might be attributed to the steric repulsion between the substituent at the terminal ring of the polycyclic phenols and the pyrenyl group of catalyst. In addition, halogen or methyl group could also be installed at the C-6 or C-9 position of substrate 1 , which appeared to be inconsequential to the reaction outcomes, delivering the desired [4]helicenes with commendable yields and enantioselectivities ( 3z - 3ab , up to 49% yield and 98:2 er). To further extend the application of the present method to the enantioselective synthesis of [5]helicenes, racemic 2-[5]helicenol 1j was recruited to undergo the current protocol. We were gratified to observe the smooth formation of 3ac in 44% yield, albeit with relatively lower er value (88:12 er). It should be noted that the recovered 1j was identified to be with an er value of 79.5:20.5, suggesting a reaction profile of catalytic kinetic resolution of configurationally unstable helical substrates at low temperature (−50 °C). Fig. 4: Substrate scope with respect to polycyclic phenols and scope of the synthesis of helicenes bearing a stereogenic C-N axis. Reaction conditions: 0.2 mmol 1 (1.0 equiv), 0.1 mmol 2 (0.5 equiv), and 5 mol% C6 in THF (1.0 mL) at −50 °C. Isolated yields based on 1 are shown. The er values were determined by HPLC analysis using a chiral stationary phase. Full size image Encouraged by the above success, we then wondered whether this approach could be utilized to construct stereochemically complex molecules, especially those with multiple stereogenic elements. To the best of our knowledge, simultaneous control of helical and other chiralities via a catalytic enantioselective process represents a formidable challenge and has rarely been reported [56] , [57] . Towards this goal, the reactions of diazodicarboxamides with a sterically bulky t -butyl group at the ortho -position of phenyl ring were further performed (Fig. 4 ), and surprisingly, supplied the respective helically chiral products bearing a stereogenic C-N axis in 45-49% yields with excellent stereoselectivities ( 3ad - 3af, 3ah and 3ai , 96.5:3.5-97.5:2.5 er, >20:1 dr). Remarkably, stereochemically complex [5]- and [6]-helicenes were also achievable with comparably high er values ( 3aj and 3ak ). 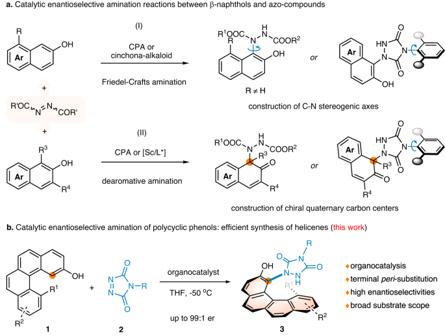Fig. 2: Diverse synthesis of compounds with different chiralities via catalytic enantioselective amination reactions of polycyclic phenols. aPrevious works: construction of axially and centrally chiral compounds by Friedel-Crafts and dearomative aminations.bThis work: construction of helically chiral molecules by developing a terminalperi-amination strategy. CPA chiral phosphoric acid. 3ag bearing a 2-iodo-6-methylphenyl ring that is found frequently in C-N axially chiral atropisomers failed to form a configurationally stable C-N axis, mainly because the intramolecular steric repulsion caused by the terminal ring of [4]helicene facilitates the axial rotation. The capacity of realizing remote axial enantiocontrol while controlling helical sense selectivity again confirmed the broad generality of this catalytic enantioselective approach to derive structurally diverse helically chiral [4]-, [5]- and [6]helicenes. Synthetic applications To demonstrate the scalability and practicality of this protocol in the synthesis of helically chiral chemicals, 2.0 mmol scale preparations of [4]helicenes 3a and 3ab under standard conditions were conducted (Fig. 5a ). To our delight, the reactions proceeded smoothly and there was no obvious erosion of yield and enantioselectivity to be observed, suggesting a potential for large-scale chemical production of this method. Furthermore, some representative transformations of the helically chiral products 3a and 3ad were exhibited to further validate the synthetic value of this methodology (Fig. 5b ). For example, double methylation of 3a with iodomethane was easily realized in the presence of K 2 CO 3 at room temperature, by which a configurationally stable C-N axis was established in a diastereoselective fashion, giving [4]helicene 4a in high yield with acceptable stereoselectivity (90% yield, 6.1:1 dr, 96.5:3.5 er). The configurationally stability of C-N axes in 4a over 3a was supported by DFT calculations. C-N bond rotation in 3a shows a medium barrier of 15.4 kcal/mol, while bond rotation in 4a is kinetically unfavorable with a higher barrier of 29.5 kcal/mol, resulting from the steric hinderance of the methyl substituents. Similarly, [4]helicene 4ad bearing two stereogenic C-N axes could also be accessed. Subjecting 3a to Raney Ni catalyst under a hydrogen atmosphere, a N–N bond cleavage and subsequent intramolecular cyclization occurred to generate biaryl compound 6 in 69% yield with excellent stereoretention. Notably, the urazole ring could also be cleaved by treating 4a with KOH in isopropanol to deliver [4]helicene 5 in 51% yield. Additionally, diverse modifications of the main helical skeleton of 4ab were also exhibited. Substituents such as aryl, alkynyl, and secondary amine groups can be readily introduced at the 6-position of [4]helicene 4ab by involving Pd-catalyzed Suzuki-Miyaura, Sonogashira and Buchwald-Hartwig amination reactions, respectively. Treating 4ab with CuCN at 140 °C produced the corresponding cyanated [4]helicene 10 with a yield of 76%. Fig. 5: Reaction scale-up and products transformations. a Large-scale preparation of 3a and 3ab . b Synthetic transformations of 3a, 3ad and 4ab . Isolated yields based on the substrate are shown. Full size image Mechanistic studies The helical structure of 4ad was unambiguously demonstrated by its X-ray crystallographic analysis (Fig. 6a ), and the corresponding absolute configuration was definitely assigned to be ( M , aS , aS ) on the basis of the Flack parameter (0.07(13)). The configurations of other newly synthesized helicenes were inferred accordingly. In addition, the circular dichroism spectra of ( P , aR )- 3ad and ( M , aS )- 3ad were recorded to investigate the chiroptical properties, which display mirror images and clear Cotton effects at around 226, 242, 261, 280, 298, and 348 nm, respectively (Fig. 6b ). Then, density functional theory calculations were conducted using the M11-L functional to obtain the interconversion profiles of the two helical enantiomers of compounds 1a and 3a , respectively (Fig. 6c ). The relatively lower calculated barrier to enantiomerization for [4]helicene 1a (ΔG ǂ = 21.5 kcal/mol) revealed its configurational lability, corresponding to a half-life of 0.1 h at room temperature. In comparison, the barrier to enantiomerization for 1,12-disubstituted [4]helicene 3a is significantly high (~40 kcal/mol), arguing for the high configurational stability of the M / P -configured 3a . Fig. 6: Mechanistic studies. 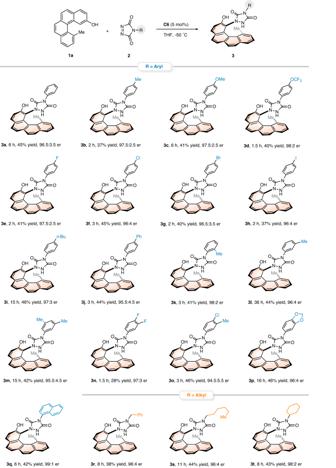Fig. 3: Substrate scope with respect to diazodicarboxamides. Reaction conditions: 0.2 mmol1a(1.0 equiv), 0.1 mmol2(0.5 equiv), and 5 mol%C6in THF (1.0 mL) at −50 °C. Isolated yields based on1aare shown. The er values were determined by HPLC analysis using a chiral stationary phase. a X-ray structure of ( M , S , S )- 4ad . b CD spectra of ( M , S )- 3ad (1.0 × 10 −3 M) and its enantiomer ( P , R )- 3ad (1.0 × 10 −3 M) in ethanol at room temperature. c Computed enantiomerization of 1a and 3a . d DFT calculated nucleophilic addition transition states with their relative free energies (in kcal/mol) and geometrical parameters (in Å). Full size image Furthermore, based on the control experiments (Supplementary Fig. 5 ) and absolute configuration of amination products, we computationally explored the nucleophilic addition transition states of 1a to 2a to gain insight into the origin of the stereochemistry of this catalytic kinetic resolution process (Fig. 6d ). The calculations revealed that catalyst C6 brings the two reactants into close proximity via hydrogen bonding interactions and locks the relative orientation of the two substrates through their non-covalent interactions with the naphthalene skeleton and the pyrenyl substituent in the catalyst. In the most favorable transition state TS- M , the bifunctional catalyst utilizes the thiourea N-H group to stabilize the anionic nucleophile ( M )- 1a , while the alkylammonium ion acts as a Brønsted acid to activate the diazodicarboxamide 2a . The reaction with ( P )- 1a is relatively disfavored by 1.9 kcal/mol in the current catalytic system, largely due to the absence of C-H---π interactions between 1a and the pyrenyl substituent of catalyst C6 (Fig. 6d , TS- P ). Additionally, the traditional activation model with the tight alkylammonium-anionic 1a ion pair is unlikely to be involved, owing to the energy-demanding transition state TS- M’ . With the favored activation model established, we next intended to unravel the origin of C-N axial chirality induction. The optimized C-N forming TSs that give rise to the major and minor diastereoisomers of the product 3ad are shown in Fig. 7 . In the transition states TS- MS and TS- MR , the phenyl ring of the diazodicarboxamide compound 2u tends to be oriented away from the terminal ring of the polycyclic phenolate, in contrast to the arrangement observed in TS- M . Transition state TS- MS , which leads to the major ( M,S )-configured product, is more favored than TS- MR by 3.3 kcal/mol. This preference arises from the decreased steric repulsion between the tert -butyl group on 2u and the polycyclic phenolate. Fig. 7: Computational investigations on the origin of C-N axial chirality induction (energy in kcal/mol and bond lengths in Å). a C-N bond forming transition state leading to the ( M , S )-configured product. b C-N bond forming transition state leading to the ( M , R )-configured product. Full size image 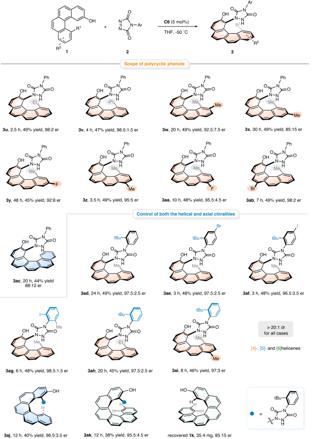Fig. 4: Substrate scope with respect to polycyclic phenols and scope of the synthesis of helicenes bearing a stereogenic C-N axis. Reaction conditions: 0.2 mmol1(1.0 equiv), 0.1 mmol2(0.5 equiv), and 5 mol%C6in THF (1.0 mL) at −50 °C. Isolated yields based on1are shown. The er values were determined by HPLC analysis using a chiral stationary phase. In conclusion, we successfully developed a terminal peri -functionalization strategy for the catalytic enantioselective preparation of helically chiral molecules. The highly enantioselective synthesis of [4]carbohelicenes has been accomplished via an organocatalyzed intermolecular electrophilic aromatic amination reaction of 2-hydroxybenzo[ c ]phenanthrene derivates with diazodicarboxamides. The capacity of simultaneous control of helical and remote C-N axial chiralities made the current protocol especially intriguing, allowing for the constructing of enantioenriched [4]-, [5]- and [6]helicenes featuring an urazole scaffold with both structural diversity and stereochemical complexity in good to excellent yields and enantioselectivities. The mechanism investigation suggests that excellent enantiocontrol stems from a catalytic kinetic resolution process of configurationally unstable polycyclic phenols under low temperature. The diverse synthesis of previously elusive optically pure helicenes based on the strategy reported herein is currently in progress. General procedure for catalytic enantioselective synthesis of 1,12-disubstituted [4]helicenes The mixture of polycyclic phenols 1 (0.2 mmol, 1.0 equiv) and catalyst C6 (0.01 mmol, 0.05 equiv) was dissolved in 1.0 mL of THF and stirred at room temperature for 10 min. Then, the solution was cooled to −50 °C and stirred for another 10 min before diazodicarboxamides 2 (0.1 mmol, 0.5 equiv) was added. 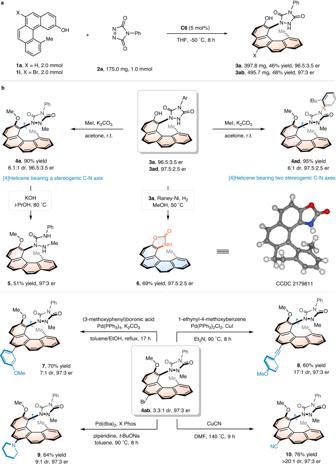Fig. 5: Reaction scale-up and products transformations. aLarge-scale preparation of3aand3ab.bSynthetic transformations of3a,3adand4ab. Isolated yields based on the substrate are shown. The resulting mixture was stirred at this temperature until the complete consumption of 2 . 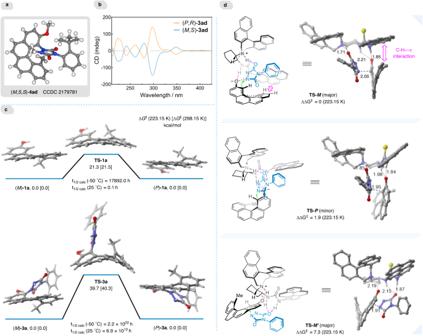Fig. 6: Mechanistic studies. aX-ray structure of (M,S,S)-4ad.bCD spectra of (M,S)-3ad(1.0 × 10−3M) and its enantiomer (P,R)-3ad(1.0 × 10−3M) in ethanol at room temperature.cComputed enantiomerization of1aand3a.dDFT calculated nucleophilic addition transition states with their relative free energies (in kcal/mol) and geometrical parameters (in Å). 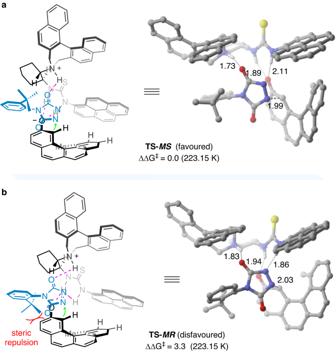Fig. 7: Computational investigations on the origin of C-N axial chirality induction (energy in kcal/mol and bond lengths in Å). aC-N bond forming transition state leading to the (M,S)-configured product.bC-N bond forming transition state leading to the (M,R)-configured product. After monitored by TLC, the solvent was removed under reduced pressure, and the residue was purified by silica gel column chromatography to afford the desired products 3 .